Tet2loss leads to hypermutagenicity in haematopoietic stem/progenitor cells TET2 is a dioxygenase that catalyses multiple steps of 5-methylcytosine oxidation. Although TET2 mutations frequently occur in various types of haematological malignancies, the mechanism by which they increase risk for these cancers remains poorly understood. Here we show that Tet2 −/− mice develop spontaneous myeloid, T- and B-cell malignancies after long latencies. Exome sequencing of Tet2 −/− tumours reveals accumulation of numerous mutations, including Apc , Nf1 , Flt3 , Cbl , Notch1 and Mll2 , which are recurrently deleted/mutated in human haematological malignancies. Single-cell-targeted sequencing of wild-type and premalignant Tet2 −/− Lin − c-Kit + cells shows higher mutation frequencies in Tet2 −/− cells. We further show that the increased mutational burden is particularly high at genomic sites that gained 5-hydroxymethylcytosine, where TET2 normally binds. Furthermore, TET2 -mutated myeloid malignancy patients have significantly more mutational events than patients with wild-type TET2 . Thus, Tet2 loss leads to hypermutagenicity in haematopoietic stem/progenitor cells, suggesting a novel TET2 loss-mediated mechanism of haematological malignancy pathogenesis. Ten eleven translocation methylcytosine dioxygenases (TET1/2/3) catalyse the conversion of 5-methylcytosine (5mC) to 5-hydroxymethylcytosine (5hmC) and can further oxidize 5hmC to 5-formylcytosine (5fC) and 5-carboxylcytosine (5caC) [1] , [2] , [3] . 5fC and 5caC can then be removed by thymine DNA glycosylase (TDG) of base excision repair (BER) [4] . Alternatively, deamination may occur at 5hmC sites by AID/APOBEC cytidine deaminases to generate 5-hydroxymethyluracil (5hmU), which can also be repaired by BER [5] . Therefore, DNA methylation and TETs/TDG-BER-driven DNA demethylation form a complete cycle of dynamic cytosine modifications. The oxidation and demethylation of 5mC in the genome are regulated in a sophisticated manner. Genetic inactivation of Tdg and Tets leads to prominent alterations of CpG modifications at various gene regulatory regions. This raises the possibility that TETs/TDG-BER-mediated cytosine modifications may be widespread across the whole genome. TET2 is one of the most commonly mutated/deleted genes in adult myeloid malignancies, including ∼ 30% of cases of myelodysplastic syndrome (MDS), 20% of myeloproliferative neoplasms (MPNs), 17% of de novo acute myeloid leukaemias (AMLs), 30% of secondary AMLs and 50–60% of chronic myelomonocytic leukaemias [6] , [7] , [8] , [9] . Somatic TET2 mutations also occur in T-cell lymphomas (such as angioimmunoblastic T lymphomas, 33%) [10] and B-cell non-Hodgkin lymphomas (diffuse large B-cell lymphoma, 12%; mantle cell lymphoma, 4%) [11] , [12] . Mutations in TET2 are also prevalent in healthy individuals over 70 years of age (>5%) and are often associated with clonal haematopoiesis [13] . These results indicate that TET2 mutations are ancestral events that drive nonmalignant clonal outgrowth and facilitate haematological malignancy transformation. Indeed, Tet2 loss in mice leads to increased haematopoietic stem cell (HSC) self-renewal and subsequent development of myeloid malignancies [14] , [15] , [16] , [17] . Loss-of-function TET2 mutations and TET2 loss result in aberrant 5mC and 5hmC profiles [14] , [18] , and we recently showed that TET2 likely requires its catalytic activity in HSC/haematopoietic progenitor cells (HPCs) to exert a tumour-suppressive function [19] . However, the mechanisms by which TET2 loss leads to diverse haematological malignancies remain largely unknown. Accumulations of mutations in HSCs/HPCs can be deleterious to haematopoietic function and promote haematological malignancy. Here we find, using our Tet2 −/− mouse models and combined biological, bioinformatics and genetic approaches, that TET2 safeguards HSCs/HPCs against genomic mutagenicity. Exome sequencing of Tet2 −/− tumours and targeted single-cell exome sequencing of premalignant wild-type (WT) and Tet2 −/− HSCs/HPCs show that TET2 loss leads to genomic hypermutability in HSCs/HPCs. We further see that Tet2 loss leads to a significantly higher mutational frequency at genomic sites that gained 5hmC on Tet2 loss, where TET2 normally binds. Our results indicate that TET2 and TET2-mediated 5 mC oxidation safeguard cells against genomic mutagenicity. These findings suggest a novel mechanism contributing to TET2 loss-mediated pathogenesis in a diverse array of haematological malignancies. Tet2 −/− mice develop myeloid and lymphoid malignancies To determine the complete spectrum of haematological malignancies caused by Tet2 loss in vivo , we conducted a 2-year follow-up study on a cohort of 198 Tet2 −/− and 67 WT mice. All Tet2 −/− mice developed spontaneous lethal haematological malignancies with survival durations ranging from 3 to 22 months, whereas no abnormalities were detected in the haematopoietic organs of WT mice ( Fig. 1a,b ). Consistent with previous observations [14] , [15] , [16] , 92% of these Tet2 −/− mice developed myeloid malignancies, as indicated by monocytosis/neutrophilia, hepatosplenomegaly and marked expansion of well-differentiated myeloid cells or erythroid precursors in the bone marrow (BM), spleen and liver ( Supplementary Fig. 1 ). Analyses of these 198 Tet2 −/− mice also showed that 3.5% of Tet2 −/− mice developed T-cell malignancies and 4.5% of Tet2 −/− mice developed B-cell malignancies ( Fig. 1b–h , Supplementary Fig. 2 and Supplementary Tables 1 and 2 ). These mice displayed marked lymphocytosis consisting of atypical lymphocytes, lymphadenopathy, hepatosplenomegaly and enlarged thymuses, in most cases with T-cell malignancies ( Fig. 1c,d ). 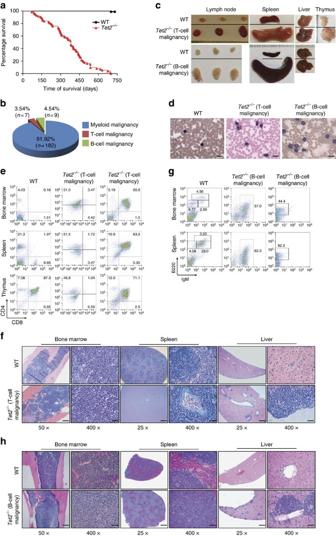Figure 1:Tet2−/−mice develop lethal lymphoid malignancies involving both T- and B-cell lineages. (a) Survival of WT (n=67) andTet2−/−(n=198) mice over time. (b) Proportions of haematological malignancy types developed in 198Tet2−/−mice. (c) Gross morphologies of lymph nodes, spleen, liver and/or thymus from representativeTet2−/−mice with T-cell (upper) or B-cell (lower) malignancy and age-matched WT mice. (d) May–Grünwald–Giemsa-stained PB smears prepared from a representative WT mouse andTet2−/−mice with T- and B-cell malignancies (scale bar, 20 μm). (e) Flow cytometric analysis of the T-cell lineage (CD4/CD8) in BM, spleen and thymus of representativeTet2−/−mice with T-cell malignancy and an age-matched WT mouse. (f) Histological analysis of H&E-stained sections of femur, spleen and liver from a representativeTet2−/−mouse with T-cell malignancy and an age-matched WT mouse (scale bar, × 25, 200 μm; × 50, 100 μm; × 400, 12.5 μm). (g) Flow cytometric analysis of the B-cell lineage (B220/IgM) in BM and spleen of representativeTet2−/−mice with B-cell malignancy and an age-matched WT mouse. (h) Histological analysis of H&E-stained sections of femur, spleen and liver from a representativeTet2−/−mouse with B-cell malignancy and an age-matched WT mouse (scale bar, × 25, 200 μm; × 50, 100 μm; × 400, 12.5 μm). Figure 1: Tet2 −/− mice develop lethal lymphoid malignancies involving both T- and B-cell lineages. ( a ) Survival of WT ( n =67) and Tet2 −/− ( n =198) mice over time. ( b ) Proportions of haematological malignancy types developed in 198 Tet2 −/− mice. ( c ) Gross morphologies of lymph nodes, spleen, liver and/or thymus from representative Tet2 −/− mice with T-cell (upper) or B-cell (lower) malignancy and age-matched WT mice. ( d ) May–Grünwald–Giemsa-stained PB smears prepared from a representative WT mouse and Tet2 −/− mice with T- and B-cell malignancies (scale bar, 20 μm). ( e ) Flow cytometric analysis of the T-cell lineage (CD4/CD8) in BM, spleen and thymus of representative Tet2 −/− mice with T-cell malignancy and an age-matched WT mouse. ( f ) Histological analysis of H&E-stained sections of femur, spleen and liver from a representative Tet2 −/− mouse with T-cell malignancy and an age-matched WT mouse (scale bar, × 25, 200 μm; × 50, 100 μm; × 400, 12.5 μm). ( g ) Flow cytometric analysis of the B-cell lineage (B220/IgM) in BM and spleen of representative Tet2 −/− mice with B-cell malignancy and an age-matched WT mouse. ( h ) Histological analysis of H&E-stained sections of femur, spleen and liver from a representative Tet2 −/− mouse with B-cell malignancy and an age-matched WT mouse (scale bar, × 25, 200 μm; × 50, 100 μm; × 400, 12.5 μm). Full size image Flow cytometric analyses of the spleen and BM cells from seven Tet2 −/− mice with T-cell malignancies revealed dominant proportions of CD3 + T lymphocytes with a high forward scatter; five of these seven animals aberrantly expressed CD4 in their T lymphocytes that were mostly positive for CD44 and PD1 ( Fig. 1e , Supplementary Fig. 2a,b and Supplementary Table 1 ). BM, spleen, liver and thymus had atypical lymphoid infiltrates effacing or distorting the normal architecture of these organs ( Fig. 1f and Supplementary Fig. 2c ). Atypical lymphocytes were medium sized, with a smaller amount of cytoplasm and irregular nuclei relative to WT. The spleen showed diffuse lymphoid infiltrates involving both red and white pulp. The liver demonstrated sinusoidal and perivascular infiltration. In addition, splenic CD3 + cells from each of the tested Tet2 −/− mice with monomorphic T-cell infiltrations showed clonal T-cell receptor rearrangement patterns ( Supplementary Fig. 2f ). In nine Tet2 −/− mice with B-cell malignancies, spleen and BM cells were dominantly B220 +/lo IgM +/lo CD19 + CD43 + TdT − B lymphocytes with a high forward scatter ( Fig. 1g , Supplementary Fig. 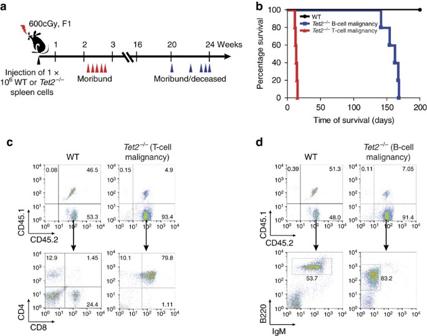Figure 2: T- and B-cell malignancies inTet2−/−mice are transplantable to sublethally irradiated secondary WT recipients. (a) Tumour transfer schema. Spleen cells (1 × 106) from representativeTet2−/−mice with a T- or B-cell malignancy or from an age-matched WT mouse were injected into sublethally irradiated (600 cGy) CD45.1+/CD45.2+F1 recipients. (b) Kaplan–Meier survival curve of sublethally irradiated recipients (five mice/donor) transplanted with spleen cells fromTet2−/−mice with T-cell (red) or B-cell (blue) malignancies or from one WT (black) mouse. (c) Flow cytometric analyses of PB T-cell lineage (CD4/CD8) donor cells (CD45.2+) from a mouse receiving spleen cells from a WT mouse or aTet2−/−mouse with T-cell malignancy. (d) Flow cytometric analyses of peripheral blood B-cell lineage (B220/IgM) donor cells (CD45.2+) from a mouse receiving spleen cells from a WT mouse or aTet2−/−mouse with B-cell malignancy. 2d and Supplementary Table 2 ). B lymphocytes from four of these mice expressed CD5 ( Supplementary Table 2 ). Neoplastic monomorphic expansions of B cells were thus observed in these Tet2 −/− mice. Atypical lymphoid infiltrates were identified in BM, spleen, liver, lymph node and small intestine ( Fig. 1h and Supplementary Fig. 2e ). Atypical lymphocytes were predominantly medium sized, with a smaller amount of cytoplasm relative to WT, and with irregular nuclear vesicular and condensed nuclear chromatin. The spleen showed effacement of normal architecture with nodular lymphoid infiltrate involving predominantly white pulp. The liver displayed perivascular and sinusoidal infiltration. The intestine showed lymphoepithelial lesions with lymphoid nodules. In addition, splenic B220 + cells from each of the tested Tet2 −/− mice with monomorphic B-cell infiltrations were clonal for IgH D–J rearrangement ( Supplementary Fig. 2g ). Lymphoid malignancies in Tet2 −/− mice are transplantable To evaluate the malignant nature of the abnormally infiltrated T and B lymphocytes in Tet2 −/− mice, spleen cells from one WT mouse and two Tet2 −/− mice with malignancies, one with a T-cell clone (G3-6) and one with a B-cell clone (G3-185), were transplanted into sublethally irradiated WT recipients ( Fig. 2a ). No recipient receiving WT spleen cells developed any evidence of disease within 6 months of transplantation ( Fig. 2b ). In contrast, all mice receiving spleen cells from Tet2 −/− mice with T- or B-cell malignancy developed diseases with characteristics similar to those observed in primary mouse, for example, elevated WBC counts, lymphocytosis, splenomegaly, enlarged lymph nodes and premature death ( Fig. 2b ). Flow cytometric analysis of peripheral blood (PB) cells of the recipients revealed infiltration of uniform, donor cell-derived, T- (CD45.2 + CD4 + CD8 + ) or B- (CD45.2 + B220 + IgM low ) cell populations, similar to what we saw in the respective primary Tet2 −/− mouse ( Fig. 2c,d ). As Tet2 −/− B- and T-cell malignancies were transplantable into sublethally irradiated WT mice, infiltrating T or B lymphocytes in these Tet2 −/− mice are indeed malignant/neoplastic. Collectively, these data demonstrate that, in addition to myeloid malignancies, Tet2 −/− mice develop lethal T- and B-cell malignancies with features most closely resembling human peripheral T-cell lymphoma not otherwise specified and acute B-lymphocytic leukaemia, respectively. These findings are consistent with clinical observations that loss-of-function mutations in TET2 are frequent in both myeloid and subtypes of B- and T-cell malignancies [6] , [7] , [8] , [9] , [10] , [11] , [16] . Figure 2: T- and B-cell malignancies in Tet2 −/− mice are transplantable to sublethally irradiated secondary WT recipients. ( a ) Tumour transfer schema. Spleen cells (1 × 10 6 ) from representative Tet2 −/− mice with a T- or B-cell malignancy or from an age-matched WT mouse were injected into sublethally irradiated (600 cGy) CD45.1 + /CD45.2 + F1 recipients. ( b ) Kaplan–Meier survival curve of sublethally irradiated recipients (five mice/donor) transplanted with spleen cells from Tet2 −/− mice with T-cell (red) or B-cell (blue) malignancies or from one WT (black) mouse. ( c ) Flow cytometric analyses of PB T-cell lineage (CD4/CD8) donor cells (CD45.2 + ) from a mouse receiving spleen cells from a WT mouse or a Tet2 −/− mouse with T-cell malignancy. ( d ) Flow cytometric analyses of peripheral blood B-cell lineage (B220/IgM) donor cells (CD45.2 + ) from a mouse receiving spleen cells from a WT mouse or a Tet2 −/− mouse with B-cell malignancy. Full size image Tet2 loss leads to hypermutagenicity in HSCs/HPCs The kinetics and the involvement of multiple lineages by haematological malignancies in Tet2 −/− mice suggest that additional genetic lesions may be acquired in these mice, resulting in the pathogenesis and/or progression of various haematological malignancies. To explore this possibility, comparative genomic hybridization arrays and whole-exome sequencing (WES) were performed using tumour and non-tumour cells from Tet2 −/− mice with myeloid, T- or B-cell malignancies. Comparative genomic hybridization arrays identified a variety of structural chromosomal abnormalities in myeloid, T- and B-cell malignancies ( Supplementary Fig. 3a and Supplementary Data 1 ). Further examination of these chromosomal deletions/gains revealed no specific regions associated with genes previously linked to tumourigenesis. WES revealed on average 10,156 nonsynonymous replacement sites and 15,809 silent sites per tumour type ( Supplementary Fig. 3b and Supplementary Data 2 ). Of the Tet2 −/− tumours of myeloid, T- or B-cell origin, we found 190 genes with recurrent single-nucleotide variants (SNVs) originating from different tumours. The gene list included Apc , Nf1 , Flt3 , Cbl , Notch1 and Mll2 ( Fig. 3a and Supplementary Data 3 ), genes recurrently altered in human haematological malignancies [20] , [21] , [22] , [23] , [24] . The heterodimerization and proline-glutamic acid-serine-threonine-rich domains of NOTCH1 are mutational hotspots in human T-ALL [24] . Notch1 mutations identified by exome sequencing and Sanger sequencing in Tet2 −/− T-cell tumours were found within these hotspots ( Fig. 3b ), suggesting that additional Notch1 mutations are acquired in Tet2 −/− mice and contribute to the initiation/progression of the T-cell malignancy. 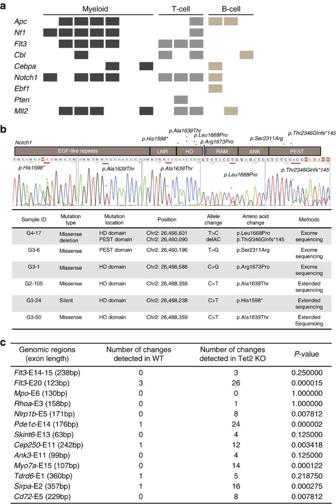Figure 3: WES reveals mutations in TET2-deficient tumours. (a) Selected recurrent gene mutations inTet2−/−tumours of myeloid, B- or T-cell lineage as identified by WES. (b)Notch1gene mutations identified by exome-sequencing and/or Sanger sequencing in sixTet2−/−T-cell tumours are summarized (lower). Sanger sequence traces of fourTet2−/−T-cell tumours with heterozygous mutations inNotch1are shown (middle). The mutational locations are shown as red asterisks in the mouse NOTCH1 protein schematic representation (upper). (c) Significantly more mutations are found in premalignantTet2−/−LK cells compared to WT LK cells by single-cell-targeted exome sequencing (Fisher’s exact test,P<0.001). Figure 3: WES reveals mutations in TET2-deficient tumours. ( a ) Selected recurrent gene mutations in Tet2 −/− tumours of myeloid, B- or T-cell lineage as identified by WES. ( b ) Notch1 gene mutations identified by exome-sequencing and/or Sanger sequencing in six Tet2 −/− T-cell tumours are summarized (lower). Sanger sequence traces of four Tet2 −/− T-cell tumours with heterozygous mutations in Notch1 are shown (middle). The mutational locations are shown as red asterisks in the mouse NOTCH1 protein schematic representation (upper). ( c ) Significantly more mutations are found in premalignant Tet2 −/− LK cells compared to WT LK cells by single-cell-targeted exome sequencing (Fisher’s exact test, P <0.001). Full size image To confirm that mutations associated with the tumours in aged Tet2 −/− mice were somatic, we performed additional WES using Lin − c-Kit + (LK) cells isolated from premalignant (6-week-old) WT, Tet2 +/− and Tet2 −/− mice. WES analyses identified few mutations in premalignant LK cells from WT, Tet2 +/− and Tet2 −/− mice, because genetic changes would only be detectable in a dominant LK cell clone ( Supplementary Data 4 ), so variants identified in Tet2 −/− tumours are somatic mutations accumulating in Tet2 −/− cells over time, rather than germline. To overcome this limitation, we performed targeted sequencing on selected loci (from the Tet2 −/− tumour SNVs) at the single-cell level using WT and premalignant Tet2 −/− LK cells. Interestingly, we observed a significantly higher frequency of mutations on seven of the 13 selected loci in Tet2 −/− LK cells compared to WT LK cells ( Fig. 3c and Supplementary Table 3 ), suggesting that Tet2 −/− LK cells are hypermutagenic. Higher mutational burden at sites with gained-5hmC peaks Given the role of TET proteins in the 5mC oxidation process, we next examined the effect of Tet2 loss on genome-wide 5hmC and 5mC modification. We applied a selective chemical labelling and affinity enrichment procedure [25] to map genome-wide 5hmC distributions in premalignant WT and Tet2 −/− LK cells ( Supplementary Data 5 ). Consistent with previous observations in mouse embryonic stem cells [26] , significant reductions of 5hmC were restricted to bodies of genes intermediately or lowly expressed in LK cells. 5hmC was not affected in highly expressed genes in Tet2 −/− LK cells ( Fig. 4a and Supplementary Fig. 4a ). Most TET2-dependent 5hmC modifications in LK cells were located within genes ( Fig. 4b ). We then explored the overlap between sites with SNVs/indels in Tet2 −/− tumours and three different genomic loci: (1) sites with no change in 5hmC/5mC peaks, presumably representing the sites with 5mC oxidation catalysed by TET1/3, but not TET2; (2) sites with 5hmC peak loss or 5mC peak gain, representing the 5mC sites that are converted to 5hmC by TET2; and (3) sites with 5hmC peak gain, likely representing the 5hmC sites that are further oxidized to 5fC/5caC by TET2 ( Fig. 4c ). Using the χ 2 test, consistent with TET2’s main role being further oxidation of 5hmC, we saw a significantly greater frequency of SNVs/indels in Tet2 −/− tumours at loci with 5hmC peak gains compared to loci with no change in 5hmC/5mC peaks and loci with 5hmC peak loss or 5mC peak gain ( Fig. 4d,e and Supplementary Fig. 4b,c ). Similar increases were also observed with C-to-T (or G-to-A) mutations ( Supplementary Fig. 4b ). This mutational occurrence at loci with 5hmC peak gain was further confirmed by traditional bisulfite sequencing and TET-assisted bisulfite sequencing at CpG sites with different distances (<30 and >100 bp) to selective mutations (detected by WES) using WT and premalignant Tet2 −/− LK cells, which showed a significantly higher percentage of CpG sites with a 5hmC gain in sites within 30 bp from the mutation sites (7 out of 10) as compared to sites >100 bp away (1 out of 10, P <0.05, by Fisher’s exact test) from the mutation sites ( Supplementary Fig. 4d,e ). Together, loci with 5hmC peak gain on Tet2 loss are associated with a higher mutational frequency. 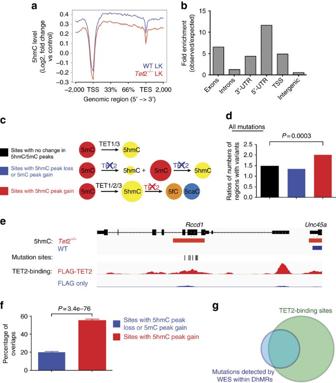Figure 4: Greater mutational frequencies at loci with 5hmC peak gains inTet2−/−tumours. (a) Distribution of average 5hmC enrichment at all genes in WT andTet2−/−LK cells. (b) Association of 5hmC-enriched regions with genomic features in LK cells. The percentage of 5hmC-enriched regions overlapping a defined genomic feature was compared to the percentage expected to fall in that particular region by chance based on the genomic coverage of that region. Values are expressed as fold change relative to expected. (c) Three categories of 5hmC loci: (1) sites with no change in 5hmC/5mC peaks, (2) sites with 5hmC peak loss or 5mC peak gain wherein TET2 was responsible for the first oxidation step and (3) sites with 5hmC peak gains wherein TET2 was responsible for the second and perhaps third oxidation steps. (d,e) Significantly greater frequencies of overall SNVs/indels inTet2−/−tumours occur within loci with 5hmC peak gains, but not in loci with no change in 5hmC/5mC peaks and loci with 5hmC peak losses or 5mC peak gains (d,P=0.0003,χ2test). Example genomic view showing overlapping features among the gained-5hmC sites onTet2loss, TET2-binding profile andRccd1mutations (e). (f) TET2 is enriched more at genomic loci with 5hmC peak gains onTet2loss (P=3.4e−76,χ2test). Error bars, s.d. (g) Venn diagram overlap between TET2-binding sites and SNVs/indels mutations associated with the loss ofTet2within DhMRs, as detected by WES. Figure 4: Greater mutational frequencies at loci with 5hmC peak gains in Tet2 −/− tumours. ( a ) Distribution of average 5hmC enrichment at all genes in WT and Tet2 −/− LK cells. ( b ) Association of 5hmC-enriched regions with genomic features in LK cells. The percentage of 5hmC-enriched regions overlapping a defined genomic feature was compared to the percentage expected to fall in that particular region by chance based on the genomic coverage of that region. Values are expressed as fold change relative to expected. ( c ) Three categories of 5hmC loci: (1) sites with no change in 5hmC/5mC peaks, (2) sites with 5hmC peak loss or 5mC peak gain wherein TET2 was responsible for the first oxidation step and (3) sites with 5hmC peak gains wherein TET2 was responsible for the second and perhaps third oxidation steps. ( d , e ) Significantly greater frequencies of overall SNVs/indels in Tet2 −/− tumours occur within loci with 5hmC peak gains, but not in loci with no change in 5hmC/5mC peaks and loci with 5hmC peak losses or 5mC peak gains ( d , P =0.0003, χ 2 test). Example genomic view showing overlapping features among the gained-5hmC sites on Tet2 loss, TET2-binding profile and Rccd1 mutations ( e ). ( f ) TET2 is enriched more at genomic loci with 5hmC peak gains on Tet2 loss ( P =3.4e−76, χ 2 test). Error bars, s.d. ( g ) Venn diagram overlap between TET2-binding sites and SNVs/indels mutations associated with the loss of Tet2 within DhMRs, as detected by WES. Full size image We next used chromatin immunoprecipitation sequencing to map genome-wide binding sites of TET2 in MEL (a mouse erythroleukaemia cell line) cells overexpressing FLAG-tagged TET2 ( Supplementary Fig. 5a,b and Supplementary Data 6 ). Genomic analysis revealed that TET2-binding sites are enriched at regions that include exons, 5′-untranslated region and CpG islands ( Supplementary Fig. 5c ). We analysed the TET2-binding sites with differentially methylated/hydroxymethylated regions in Tet2 −/− LK cells and observed significant overlap among genes involved in myeloid and B-cell differentiation ( Supplementary Fig. 5d,e ). In particular, TET2 is enriched more at loci with 5hmC peak gain on Tet2 loss ( Fig. 4f ). Furthermore, the majority of mutations we detected within loci that require TET2 for dynamic DNA demethylation overlap with TET2-binding sites ( Fig. 4g ; 145 out of 212 mutation sites). Collectively, these results suggest that TET2 binds to loci marked by a gain of 5hmC on TET2 loss, and that at these sites, TET2 may protect genome stability. TET2 loss is associated with increased mutational frequency We next examined whether TET2 loss affects the spontaneous forward mutational frequency in the hypoxanthine-guanine phosphoribosyltransferase 1 ( HPRT1 ) gene in control and TET2 kd HeLa cells. The HPRT1 mutational frequency in TET2 kd HeLa cells increased about 24-fold compared to control HeLa cells ( Fig. 5a and Supplementary Fig. 6a,b ). Similar results were obtained using control and Tet2 kd NIH3T3 cells ( Supplementary Fig. 6c,d ). When we stably re-expressed TET2 using a lentiviral construct containing a mammalian codon-optimized cDNA sequence of TET2 into TET2 kd HeLa cells ( Supplementary Fig. 6e ), HPRT1 mutational frequencies were completely rescued ( Fig. 5a ). These results indicate that TET2 loss causes increases in mutation rates. We then analysed the spectrum of mutations identified in the HPRT1 gene in 6-thioguanine (6-TG)-resistant clones of TET2 kd HeLa cells. Interestingly, SNVs and single-nucleotide insertions/deletions (indels) dominated the mutations in the HPRT1 gene. Approximately 61% and 36% of the mutations in TET2 kd clones were transitions and transversions, respectively, and ∼ 3% were indels ( Supplementary Fig. 6f ). We further analysed the mutational spectrum of Tet2 −/− tumours. We focussed on mutations located at loci with 5hmC peak gains. Base transition mutations clearly dominated the mutational spectrum in Tet2 −/− tumours, with G:C to A:T transitions accounting for 35% of total mutations. The remaining mutations consisted primarily of A:T to G:C transitions (23%), various transversions (38%), with G:C to T:A being the most frequent, and +1/−1 indels (4%), with −1 deletions being more common than +1 ( Fig. 5b ). Of all mutations isolated, 73% occurred at CpG sites or clustered around CpG sites (±30 bp); since the average distance between CpG sites across the genome is 100 bp [27] , [28] , <60% was expected in the gene bodies. The close association of mutation sites with CpG sites suggests a preference of mutational occurrence at or around CpG sites in Tet2 −/− tumours. The hypermutagenicity and mutational spectra of TET2 kd and Tet2 −/− cells and the function of TET2/TDG in 5mC oxidation and demethylation suggest that TET2 is likely involved in safeguarding genomic mutagenicity. 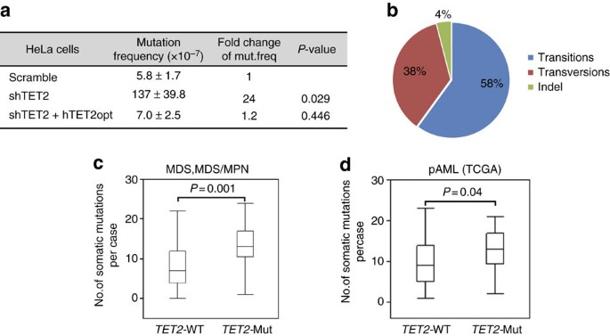Figure 5:TET2loss/mutations are associated with increased mutational frequency and specific mutational spectra. (a)HPRTmutations in scrambled control-, shTET2- and shTET2+TET2opt HeLa cells. (b) Proportions ofTet2−/−tumour transitions, transversions and indels. (c) Comparison of numbers of nonsynonymous somatic mutations by WES MDS and MDS/MPN cases with (n=41) and without (n=154)TET2mutations (P=0.001, Wilcoxon’s rank-sum test). (d) Comparison of numbers of nonsynonymous somatic mutations in AML cases with and withoutTET2mutations (P=0.04, Wilcoxon’s rank-sum test) available only for primary AMLs through TCGA. Box plots: upper whisker, maximum value less than 75%+1.5 × IQR; upper box end, 75%; bar, 50%; lower box end, 25%; lower whisker, least value more than 25%−1. × IQR. IQR, interquartile range. Figure 5: TET2 loss/mutations are associated with increased mutational frequency and specific mutational spectra. ( a ) HPRT mutations in scrambled control-, shTET2- and shTET2+TET2opt HeLa cells. ( b ) Proportions of Tet2 −/− tumour transitions, transversions and indels. ( c ) Comparison of numbers of nonsynonymous somatic mutations by WES MDS and MDS/MPN cases with ( n =41) and without ( n =154) TET2 mutations ( P =0.001, Wilcoxon’s rank-sum test). ( d ) Comparison of numbers of nonsynonymous somatic mutations in AML cases with and without TET2 mutations ( P =0.04, Wilcoxon’s rank-sum test) available only for primary AMLs through TCGA. Box plots: upper whisker, maximum value less than 75%+1.5 × IQR; upper box end, 75%; bar, 50%; lower box end, 25%; lower whisker, least value more than 25%−1. × IQR. IQR, interquartile range. Full size image We further analysed a large cohort of MDS and MDS/MPN patients ( Supplementary Table 4 ) for the presence of somatic mutations using exome sequencing of paired samples and targeted deep sequencing of 60 genes (including TET2 ) commonly mutated in these conditions ( Supplementary Data 7 ). Exome analysis revealed that patients with TET2 mutations harbour a significantly higher number of mutational events compared to those with WT TET2 ( Fig. 5c ). Similar results were obtained in AML patient data when the The Cancer Genome Atlas (TCGA) leukaemia cohort was analysed ( Fig. 5d ). Of the 556 mutations identified in MDS and MDS/MPN patients with TET2 mutations, 52% and 12% were transitions and indels, respectively ( Supplementary Fig. 6g ), slightly higher than in patients with WT TET2 ( Supplementary Fig. 6h ). Confirmatory deep sequencing of a combined cohort showed that somatic TET2 mutations were associated with other subclonal events, chiefly in APC , NF1 , ASXL1 , CBL and ZRSR2 . Consistently, many of these genes (for example, Apc , Nf1 and Cbl ) are also affected by subclonal mutations in Tet2 −/− mice ( Fig. 3a ). Increases in numbers of subclonal events in patients with TET2 mutations are consistent with Tet2 loss leading to genome-wide hypermutability in HSCs/HPCs. In this study we show that, in addition to myeloid malignancies, a fraction of Tet2 −/− mice develop T- and B-cell malignancies. These findings are consistent with clinical observations that loss-of-function mutations in TET2 arise not only in human myeloid malignancies but also in subtypes of B- and T-cell malignancies [6] , [7] , [8] , [9] , [10] , [11] , [16] . Therefore, our Tet2 −/− mice can serve as a model for investigations of mechanisms by which Tet2 loss leads to diverse haematological malignancies. Leukaemogenesis is a multistep process of acquiring gene mutations. Loss-of-function TET2 mutations are initiating events in the pathogenesis of haematological malignancies. The occurrence of secondary oncogenic gene mutations, presumably in an early haematopoietic progenitor, is likely capable of modifying the disease phenotype and/or promoting the transformation/progression of a specific haematological malignancy in Tet2 −/− mice. WES identified numerous SNVs/indels in Tet2 −/− tumours, indicating that TET2 loss constitutes a state of genetic mutagenicity. Consistently, the number of mutational events appears to be higher in MDS, MDS/MPN and primary AML patients harbouring TET2 mutations compared to those with WT TET2 . However, this observation from patient exome analysis does not necessarily imply a direct role of TET2 mutations in promoting additional mutations, since other factors associated with patients with TET2 mutations might also contribute to this observation such as older ages, increased stem cell proliferation and/or longer average disease latency due to a preceding phase of clonal haematopoiesis. The increased susceptibility to mutation acquisitions is likely further accelerated in TET2- deficient HSCs/HPCs since Tet2 loss induced intrinsic changes in these cells, with increased self-renewal and proliferation. Our study identified mutations on the genes implicated in the pathogenesis of the diverse disease phenotypes in Tet2 −/− mice. Mutations in Notch1 , Flt3 , Nf1 , Ebf1 , Apc , Cbl and other genes in the Tet2 −/− haematological malignancies are consistent with human haematological malignancy gene alterations [20] , [21] , [22] , [23] , [24] . Recent studies have shown that TET2 mutations also occur in healthy elderly individuals with clonal haematopoiesis [13] . Therefore, as an ancestral event in haematological malignancies and elderly individuals, TET2 mutations represent a suitable target for intervention at the early stages of clonal expansion of HSCs/HPCs. Although we have shown that the catalytic activity of TET2 is essential for its myeloid tumour-suppressive function in HSCs/HPCs [19] , our recent RNA-seq and 5mC/5hmC analyses on premalignant Tet2 −/− and WT LK cells showed that distinct cytosine modifications (particularly 5hmC) often mark specific genes in Tet2 −/− LK cells without altering their expression [17] . The oxidation and demethylation of 5mC in the genome are regulated in a sophisticated manner. 5fC and 5caC are substrates for TDG [1] , [29] . TETs and TDG initiate active DNA demethylation by oxidation of 5mC and excision of 5fC/5caC in DNA, followed by incision and repair of the resulting abasic site (AP site). Although the BER process is highly accurate, errors may occur due to replication across 5mC derivatives and due to polymerase errors during gap filling. Indeed, a recent in vitro biochemical study showed that TET1 and TDG mediate sequential demethylation of symmetrically methylated CpGs to avoid DNA double-strand breaks, which could kill or transform the cells [30] . 5mC is found to be a mutagen in tumour cells [31] . In addition, a recent report finds that ‘G’-5caC base pairs mimic mismatches during DNA replication [32] . Thus, genomic 5mC derivatives should normally be processed error free by BER, with mismatch repair likely serving as a ‘backup’ for certain 5mC oxidation derivatives during DNA replication. Mutations are generally considered to occur randomly throughout the genome. Although we did not observe an overt base preference in Tet2 −/− tumours mutations, the mutations did tend to be proximal to CpG sites. Our study also demonstrated that a significantly higher frequency of mutations occurred at loci with the gain of 5hmC in Tet2 −/− tumours, where TET2 normally binds. The mechanisms that govern the association of Tet2 loss with increased local mutation rates at/around gained-5hmC sites remain to be determined. A recent study showed that Ung −/− mice exhibit higher spontaneous mutation rates and increases in spontaneous B-cell lymphomas [33] . Furthermore, Mbd4 −/− mice were recently characterized as having increased rates of C-to-T transitions at CpG sites [34] . In this backdrop, our studies suggest that TET2 loss and TET2 loss-mediated 5mC oxidation dysregulation are associated with increased mutagenicity at specific genomic loci. Thus, TET2 protects HSC/HPC genomes against mutagenicity. There are now genomic profiling methods for 5fC and 5caC [35] , [36] , [37] . Given that 5fC and 5caC are directly excised by TDG/BER during active demethylation, it will be interesting to see whether sites with alterations in 5fC and 5caC marks in Tet2 −/− LK cells are preferentially associated with higher mutation rates. Parallel, genome-wide, base-resolution maps of 5mC, 5hmC, 5fC and 5caC in Tet2 −/− and WT LK cells are warranted for dissecting TET2-mediated genome-wide DNA demethylation dynamics in HSCs/HPCs and for uncovering correlations between specific 5mC, 5hmC, 5fC or 5caC alterations and the genomic hypermutagenicity caused by Tet2 loss. Indeed, consistent with our results, a recent report provides evidence that, more than TET1 or 3, a forte of TET2 is the further oxidation of 5hmC [38] . In summary, we show that TET2 loss leads to hypermutagenicity in HSCs/HPCs, preferentially at loci with the gain of 5hmC on the loss of TET2, where TET2 normally binds. TET2-dependent 5hmC marks are highly enriched at gene bodies, such as exons of LK cells. TET2 -deficient HSCs/HPCs that become hypermutagenic are likely not malignant per se , but higher mutation rates in these cells may result in additional driver mutation(s) in TET2 target genes over time. Such states may be amenable to TET2 activity-boosting chemoprevention approaches. Our results unveil a novel role for TET2 in safeguarding genome mutagenicity and provide additional insights into the mechanisms by which loss-of-function TET2 mutations cause diverse human haematological malignancies. Further mechanistic studies are needed to determine how TET2 loss leads to increased DNA mutagenicity in HSCs/HPCs and thus the increased risks of haematopoietic malignancies. Analyses of mice Tet2 -knockout ( Tet2 −/− ) mice were generated as described [14] . Animal care was conducted in accordance with institutional guidelines and approved by the Institutional Animal Care and Use Committee (IACUC), University of Miami Miller School of Medicine. PB was collected by retro-orbital bleeding of mice and was smeared for May–Grünwald–Giemsa staining, and/or subjected to an automated blood count (Hemavet System 950FS). For histopathology analyses, femurs were fixed in formaldehyde, decalcified and paraffin embedded. Spleens, livers, lymph nodes, thymus and intestine were treated similarly, except for the decalcification step. Sections (4.5 μm) were stained with haematoxylin and eosin (H&E). For flow cytometric analyses, single-cell suspensions from BM, spleen, liver, lymph node, thymus and PB were stained with panels of fluorochrome-conjugated antibodies. Dead cells were excluded by 4,6-diamidino-2-phenylindole staining. Analyses were performed using a BD FACSCanto II or LSRII flow cytometer. All data were analysed by FlowJo7.6 software. Mouse exome sequencing Initial WES was carried out to identify candidate mutations in the exome of genes. Genomic DNA was captured with the NimbleGen mouse exome array according to the manufacturer’s protocol, and 100-bp paired-end sequencing was performed using an Illumina HiSeq 2000. Raw sequencing reads were mapped to the whole mouse genome (mm10) using PEMapper/PECaller ( https://github.com/wingolab-org/pecaller ) with the default settings [39] , and variant bases were annotated with SeqAnt ( http://seqant.genetics.emory.edu/ ) [40] . For samples subjected to mutation detection, genomic DNA was amplified in selected exons by PCR (primers shown in Supplementary Data 8 ) and sequenced by Sanger sequencing. The location and types of mutations were then determined by sequencing results. HPRT mutation analyses Mutation analyses can be achieved in proliferating cells in vitro by anHPRT1 assay that positively selects for HPRT-deficient mutants based on their resistance to 6-TG, which is lethal to HPRT-WT cells that are proficient in free purine base salvage [41] . The HPRT mutation assay was conducted as described previously [42] . Briefly, cells (5 × 10 5 ) were seeded in triplicate in 10-cm petri dishes for 12 h and fed with complete medium containing 5 μM freshly prepared 6-TG. Plating efficiency was determined by culturing 5 × 10 2 cells in the absence of 6-TG. After 10 days of culturing, colonies were visualized by staining with 0.05% crystal violet. The mutation frequency was then the ratio of the number of clones in the presence of 6-TG to the total number of cells plated, normalized by the plating efficiency. Types of mutations were characterized by DNA sequencing coding regions of the HPRT gene using primers shown in Supplementary Data 8 . Patients The mutational statuses for TET2 and other coexisting genes were analysed in BM and blood specimens from patients with various myeloid neoplasms, including MDS, MDS/MPN and secondary AML (see Supplementary Table 4 and Supplementary Data 5 ). Informed consent was obtained according to protocols approved by the institutional review boards and in accordance with the Declaration of Helsinki. Diagnosis was confirmed at each institution according to the World Health Organization classification criteria. Analysis of TCGA primary AML cases was performed using publically available data sets ( http://tcga-data.nci.nih.gov/tcga/tcgaHome2.jsp ). WES for human patient samples WES and targeted capture sequencing were performed as described previously [43] . For WES, the 50 Mb of protein coding sequences was enriched from total genomic DNA by liquid-phase hybridization using SureSelect (version 4) (Agilent Technology), followed by massively parallel sequencing with HiSequation 2000 (Illumina). Somatic mutations were detected using our in-house pipeline, followed by validation using amplicon deep sequencing [43] , [44] . To minimize false positives and focus on the most prevalent or relevant somatic events, we implemented a rational bioanalytic filtering approach and applied heuristic bioanalytic pipelines. We used two independent pipelines to identify somatic and germline alterations. For confirmation of somatic mutations, we analysed paired germline DNA from CD3 + lymphocytes. The selected observations were validated by targeted deep sequencing using MiSeq. Our sequence library for deep sequencing was generated by TruSeqCustom Amplicon (Illumina). Targeted multiamplicon deep sequencing of patient samples We applied multiamplicon-targeted deep sequencing (TrueSeq; Illumina) to frequently affected exons of 60 selected genes [45] . The sequencing libraries were generated according to an Illumina paired-end library protocol and subjected to deep sequencing on MiSeq (Illumina) instrumentation according to standard protocol. High-probability oncogenic mutations were called by eliminating sequencing/mapping errors and known/possible single-nucleotide polymorphisms based on available databases and frequencies of variant reads. Genomic copy number status was calculated by directly enumerating corresponding sequencing reads in each exon. Statistical analysis Differences between experimental groups were determined by the Student’s t -test, Fisher’s exact test, Wilcoxon’s rank-sum test and/or analysis of variance, followed by Newman–Keuls multiple comparison tests as appropriate. P values <0.05 were considered significant. For SNV count data, χ 2 tests were used as implemented in R ( http://cran.r-project.org/ ) 46 . Data availability Genome-wide data sets generated for this study are deposited at GEO under the accession number GSE74390. All other remaining data are available within the article and Supplementary Files , or available from the authors on request. How to cite this article: Pan, F. et al. Tet2 loss leads to hypermutagenicity in haematopoietic stem/progenitor cells. Nat. Commun. 8, 15102 doi: 10.1038/ncomms15102 (2017). Publisher’s note: Springer Nature remains neutral with regard to jurisdictional claims in published maps and institutional affiliations.